Designing a practical high-fidelity long-time quantum memory Quantum memory is a central component for quantum information processing devices, and will be required to provide high-fidelity storage of arbitrary states, long storage times and small access latencies. Despite growing interest in applying physical-layer error-suppression strategies to boost fidelities, it has not previously been possible to meet such competing demands with a single approach. Here we use an experimentally validated theoretical framework to identify periodic repetition of a high-order dynamical decoupling sequence as a systematic strategy to meet these challenges. We provide analytic bounds—validated by numerical calculations—on the characteristics of the relevant control sequences and show that a ‘stroboscopic saturation’ of coherence, or coherence plateau, can be engineered, even in the presence of experimental imperfection. This permits high-fidelity storage for times that can be exceptionally long, meaning that our device-independent results should prove instrumental in producing practically useful quantum technologies. Developing techniques for the preservation of arbitrary quantum states—that is, quantum memory—in realistic, noisy physical systems is vital if we are to bring quantum-enabled applications including secure communications and quantum computation to reality. Although numerous techniques relying on both open- and closed-loop control have been devised to address this challenge, dynamical error suppression strategies based on dynamical decoupling (DD) [1] , [2] , [3] , [4] , dynamically corrected gates (DCGs) [5] , [6] and composite pulsing [7] are emerging as a method of choice for physical-layer decoherence control in realistic settings described by non-Markovian open-quantum-system dynamics. Theoretical and experimental studies in a variety of platforms [8] , [9] , [10] , [11] , [12] , [13] , [14] , [15] , [16] , [17] , [18] , [19] , [20] , [21] , [22] , [23] have consistently pointed to dynamical error suppression as a resource-efficient approach to substantially reducing physical error rates. Despite these impressive advances, investigations to date have largely failed to capture the typical operating conditions of any true quantum memory; namely, high-fidelity storage of quantum information for arbitrarily long-storage times, with on-demand access. This would be required, for instance, in a quantum repeater, or in a quantum computer where some quantum information must be maintained with error rates deep below fault-tolerant thresholds while large blocks of an algorithm are carried out on other qubits. Instead, both experiment and theory have primarily focused on two control regimes [24] : the ‘coherence-time regime,’ where the goal is to extend the characteristic (‘1/ e ’ or T 2 ) decay time for coherence as long as possible, and the ‘high-fidelity regime,’ where the goal is to suppress errors as low as possible for storage times short compared with T 2 (for instance, during a single gating period). Similarly, practical constraints on control timing and access latency—of key importance to laboratory applications—have yet to be considered in a systematic way. In this Article, we demonstrate how to realize a practically useful quantum memory via dynamical error suppression. Specifically, our studies identify the periodic repetition of a high-order DD sequence as an effective strategy for memory applications, considering realistic noise models, incorporating essential experimental limitations on available controls, and addressing the key architectural constraint of maintaining short access latencies to stored quantum information. We consider a scenario where independent qubits couple to a noisy environment, and both dephasing and depolarization errors introduced by realistic DD sequences of bounded-strength π -pulses are fully accounted for. We analytically and numerically characterize the achievable long-time coherence for repeated sequences and identify conditions under which a stroboscopic ‘coherence plateau’ can be engineered, and fidelity guaranteed to a desired level at long-storage times—even in the presence of experimentally realistic constraints and imperfections. We expect that our approach will provide a practical avenue to high-fidelity low-latency quantum storage in realistic devices. Model The salient features of our approach may be appreciated by first focusing on a single-qubit subject to dephasing. In the absence of control, we consider a model Hamiltonian of the form , where the Pauli matrix σ z and 0 define the qubit quantization axis and internal energy, respectively (we can set 0 =0 henceforth), and B z , H E are operators acting on the environment Hilbert space. An exact analysis of both the free and the controlled dynamics is possible if the environment can be described in terms of either a quantum bosonic bath in thermal equilibrium (spin-boson model), a weakly-coupled quantum spin bath (spin-bath model), or a stationary Gaussian stochastic process (classical-noise model) [1] , [4] , [25] , [26] , [27] , [28] , [29] , [30] , [31] . Such dephasing models provide an accurate physical description whenever relaxation processes associated with energy exchange occur over a characteristic time scale ( T 1 ) substantially longer than any typical time scale associated with the dephasing dynamics. As a result, our analysis is directly relevant to a wide range of experimentally relevant qubit systems, from trapped ions and atomic ensembles [8] , [10] to spin qubits in nuclear and electron magnetic resonance and quantum dots [12] , [13] , [14] , [17] , [31] , [32] . We shall proceed by considering the effects of DD within a filter-design framework, which generalizes the transfer-function approach widely used across the engineering community [33] and provides a transparent and experimentally relevant picture of the controlled dynamics in the frequency domain [8] , [9] , [24] , [26] , [34] , [35] . In order to more easily introduce key concepts and clearly reveal our underlying strategy, we first consider an idealized ‘bang–bang’ DD setting in which perfect instantaneous π rotations are effected by using unbounded control amplitudes. As we move forward, we will relax these unphysical constraints, and demonstrate how similar results may be obtained with experimentally realistic controls. In such an idealized control scenario, a DD sequence may be specified in terms of the pulse-timing pattern , where we also define t 0 ≡0, t n +1 ≡ T p as the sequence duration, and we take all the interpulse intervals ( t j +1 − t j ) to be lower-bounded by a minimum interval τ (ref. 28 ). The control propagator reads , with y p ( t ) being a piecewise-constant function that switches between ±1 whenever a pulse is applied. The effect of DD on qubit dephasing may be evaluated exactly in terms of a spectral overlap of the control modulation and the noise power spectral density, S ( ω ) (refs 26 , 34 ), which is determined by the Fourier transform of the two-time noise correlation function [30] . Typically, S ( ω ) has a power-law behaviour at low frequencies, and decays to zero beyond an upper cutoff ω c , that is, S ( ω ) ∝ ω s f ( ω , ω c ), and the ‘rolloff function’ f specifies the high-frequency behaviour, f =Θ( ω − ω c ) corresponding to a ‘hard’ cutoff. Let denote the Fourier transform of y p ( t ), which is given by (refs 4 , 26 ). The filter function (FF) of the sequence p is given by , and the bang–bang-controlled qubit coherence decays as e - χ p , where the decoupling error at time t = T p , and the case n =0 recovers free evolution over [0, T p ]. In this framework, the applied DD sequence behaves like a ‘high-pass’ filter, suppressing errors arising from slowly fluctuating (low-frequency) noise. Appropriate construction of the sequence then permits the bulk of the noise power spectrum to be efficiently suppressed, and coherence preserved. For a given sequence p , this effect is captured quantitatively through the order of error suppression α p , determined by the scaling of the FF near ω =0, that is, , for a sequence-dependent pre-factor A bb . A high multiplicity of the zero at ω =0 leads to a perturbatively small value of χ p as long as ω c . In principle, one may thus achieve low-error probabilities over a desired storage time T s simply by using a high-order DD sequence, such as concatenated DD (CDD; ref. 3 ), or Uhrig DD (UDD; ref. 4 ), with the desired storage time T s ≡ T p . Quantum memory requirements Once we attempt to move beyond this idealized scenario in order to meet the needs of a practically useful, long-time quantum memory, several linked issues arise. First, perturbative DD sequences are not generally viable for high-fidelity long-time storage as they require arbitrarily fast control ( τ →0). Real systems face systematic constraints mandating τ >0, and as a result, increasing α p necessitates extension of T p , placing an upper bound on high-fidelity storage times [27] , [28] , [36] . (For instance, a UDD n sequence achieves α p = n with n pulses, applied at .) For fixed T p , increasing α p implies increasing n , at the expense of shrinking τ as τ ≡ t 1 = O ( T p / n 2 ). If τ >0 is fixed, and α p is increased by lengthening T p , eventually the perturbative corrections catch up, preventing further error reduction. Second, potentially useful numerical DD approaches, such as randomized DD [37] , [38] or optimized ‘bandwidth-adapted’ DD [28] , become impractical as the configuration space of all possible DD sequences over which to search grows exponentially with T s . Third, DD exploits interference pathways between control-modulated trajectories, meaning that mid-sequence interruption ( t < T p ) typically result in significantly sub-optimal performance ( Fig. 1 ). However, a stored quantum state in a practical quantum memory must be accessible not just at a designated final retrieval time but at intermediate times also, at which it may serve as an input to a quantum protocol. 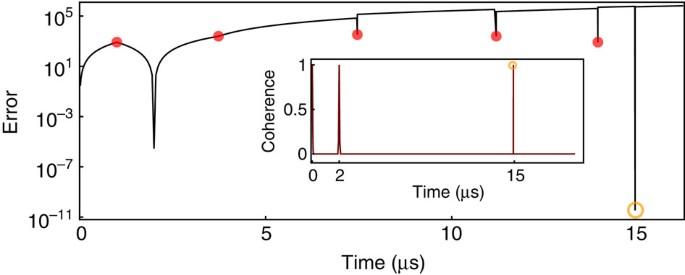Figure 1: Access latency in high-order DD sequences. DD error and coherence (inset) during a UDD5sequence with minimum interpulse timeτ=1 μs. Pulse times are marked with filled circles while the open circle indicates the readout timeTp. Minimal error (maximal coherence) is reached only at the conclusion of the sequence, with the coherence spike near 2 μs resulting from a spin–echo effect. For illustration purpose, in all figures we assume a phenomenological noise model appropriate for nuclear-spin-induced decoherence in a spin qubit in GaAs,, withω[ωmin,ωmax]. We setg=0.207ωc,ωc/2π=10 kHz,ωmin/2π=0.01 Hz, andωmax/2π=108Hz to maximize agreement with the measuredT2(≈35 ns)13,44. We choseτwell above technological constraints (~ns) in order to reducen. Figure 1: Access latency in high-order DD sequences. DD error and coherence (inset) during a UDD 5 sequence with minimum interpulse time τ =1 μs. Pulse times are marked with filled circles while the open circle indicates the readout time T p . Minimal error (maximal coherence) is reached only at the conclusion of the sequence, with the coherence spike near 2 μs resulting from a spin–echo effect. For illustration purpose, in all figures we assume a phenomenological noise model appropriate for nuclear-spin-induced decoherence in a spin qubit in GaAs, , with ω [ ω min , ω max ]. We set g =0.207 ω c , ω c /2 π =10 kHz, ω min /2 π =0.01 Hz, and ω max /2 π =10 8 Hz to maximize agreement with the measured T 2 (≈35 ns) [13] , [44] . We chose τ well above technological constraints (~ns) in order to reduce n . Full size image Addressing all such issues requires a systematic approach to DD sequence construction. Here, we identify a ‘modular’ approach to generate low-error, low-latency DD sequences for long-time storage out of shorter blocks: periodic repetition of a base, high-order DD cycle. Quantum memory via periodic repetition The effect of repetition for an arbitrary sequence is revealed by considering the transformation properties of the FF under sequence combination. Consider two sequences, p 1 and p 2 , joined to form a longer one, denoted p 1 + p 2 , with propagator y p 1 + p 2 ( t ). In the Fourier space we have Let now [ p ] m denote the sequence resulting from repeating p , of duration T p , m times, with T s = mT p . Computing by iteration, the following exact expression is found: Equation (1) describes dephasing dynamics under arbitrary multipulse control, generalizing special cases in which this strategy is implicitly used for simple base sequences (periodic DD, p ={ τ , τ } (ref. 27 ) and Carr–Purcell, p ={ τ , 2 τ , τ }), and showing similarities with the intensity pattern due to an m -line diffraction grating [31] . The single-cycle FF, F p ( ω ), is multiplied by a factor that is rapidly oscillating for large m and develops peaks scaling with at multiples of the ‘resonance frequency,’ ω res =2 π / T p , introduced by the periodic modulation (see Fig. 2 for an illustration). 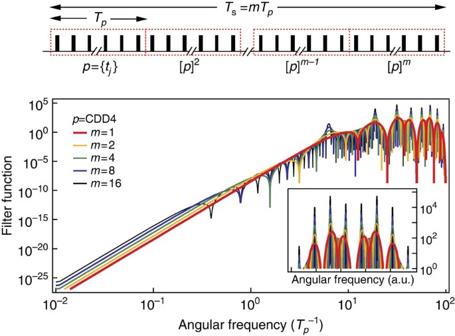Figure 2: Schematic representation of base sequence repetition and the effect on the FF. Top: The base sequencepis indicated in red dashed boxes, and repeatedmtimes up to a total storage timeTs. Bottom: FF for repetition of a CDD4cycle. The FF on a log–log plot grows with frequency with slope set byαpuntil it reaches the passband, where noise is passed largely unimpeded (red thick line). Noise dominated by spectral components in this region is efficiently suppressed by DD. Asmgrows, the sinusoidal terms in Equation (1) lead to the emergence of ‘resonance’ frequencies that modify the single-cycle FF and produce sharp peaks in the passband. These must be considered when accounting for the effects of noise at long-storage time due to ‘resonance’ effects. Inset: FF passband on a log-linear plot. Figure 2: Schematic representation of base sequence repetition and the effect on the FF. Top: The base sequence p is indicated in red dashed boxes, and repeated m times up to a total storage time T s . Bottom: FF for repetition of a CDD 4 cycle. The FF on a log–log plot grows with frequency with slope set by α p until it reaches the passband, where noise is passed largely unimpeded (red thick line). Noise dominated by spectral components in this region is efficiently suppressed by DD. As m grows, the sinusoidal terms in Equation (1) lead to the emergence of ‘resonance’ frequencies that modify the single-cycle FF and produce sharp peaks in the passband. These must be considered when accounting for the effects of noise at long-storage time due to ‘resonance’ effects. Inset: FF passband on a log-linear plot. Full size image After many repeats, the DD error is determined by the interplay between the order of error suppression of the base sequence, the noise power behaviour at low frequencies and the size of noise contributions at the resonance frequencies. The case of a hard upper frequency cutoff at ω c is the simplest to analyse. Applying the Riemann–Lebesgue lemma removes the oscillating factor, resulting in the following asymptotic expression: provided that χ [ p ] ∞ is finite. The meaning of this exact result is remarkable: for small m , the DD error initially increases as ( m 2 χ p ), until coherence stroboscopically saturates to a non-zero residual plateau value ( ), and no further decoherence occurs. Mathematically, the emergence of this coherence plateau requires that simple conditions be obeyed by the chosen base sequence relative to the characteristics of the noise: which correspond to removing the singularity of the integrand in equation (2) at 0 and ω res , respectively. Thus, judicious selection of a base sequence, fixing α p and T p , can guarantee indefinite saturation of coherence in principle. Moreover, as for all m , the emergence of coherence saturation in the infinite-time limit stroboscopically guarantees high-fidelity throughout long-storage times. By construction, this approach also guarantees that access latency is capped at the duration of the base sequence, with ; sequence interrupts at intermediate times that are multiples of T p are thus permitted in the plateau regime without degradation of error suppression. Additional insight into the above phenomenon may be gained by recalling that for free dephasing dynamics ( α p =0), the possibility of non-zero asymptotic coherence is known to occur for supra-Ohmic ( s >1) bosonic environments [25] , [27] , consistent with equation (3). The onset of a plateau regime in the controlled dynamics may then be given an intuitive interpretation by generalizing the analysis carried out in Hodgson et al. [27] for periodic DD: if the conditions in equation (3) are obeyed, the low-frequency (long-time) behaviour becomes effectively supra-ohmic by action of the applied DD sequence and, after a short-time transient, the dephasing dynamics ‘oscillate in phase’ with the periodically repeated blocks. For sufficiently small T p , the ‘differential’ DD error accumulated over each cycle in this steady state is very small, leading to the stroboscopic plateau. Interestingly, that phase noise of a local oscillator can saturate at long times under suitable spectral conditions has also long been appreciated in the precision oscillator community [33] . In light of the above considerations, the occurrence of a coherence plateau may be observed even for sub-Ohmic noise spectra ( s <1), as typically encountered, for instance, in both spin qubits ( s =−2, as in Fig. 1 ) and trapped ions ( s =−1, see ref. 39 ). Numerical calculations of the DD error using such realistic noise spectra demonstrate both the plateau phenomenon and the natural emergence of periodically repeated sequences as an efficient solution for long-time storage, also confirming the intuitive picture given above. In these calculations, we employ a direct bandwidth-adapted DD search up to time T s , by enforcing additional sequencing constraints. Specifically, we turn to Walsh DD, wherein pulse patterns are given by the Walsh functions, to provide solutions that are efficient in the complexity of sequencing [29] . Walsh DD comprises familiar DD protocols, such as spin echo, Carr–Purcell and CDD, along with more general protocols, including repetitions of shorter sequences. Starting with a free evolution of duration τ , all possible Walsh DD sequences can be recursively built out of simpler ones within Walsh DD, doubling in length with each step. Further, as all interpulse intervals in Walsh DD protocols are constrained to be integer multiples of τ , there are Walsh DD sequences that stop at time T s , a very small subset of all possible digital sequences, enabling an otherwise intractable bandwidth-adapted DD numerical minimization of the spectral overlap integral . Representative results are shown in Fig. 3 , where for each T s all Walsh DD sequences with given τ are evaluated and those with the lowest error are selected. The choice of τ sets the minimum achievable error and also determines whether a plateau is achievable, as, for a given T s , it influences the available values of T p and α p . As T s grows, the best performing sequences (shown) are found to consist of a few concatenation steps (increasing α p of the base sequence to obey equation (3)), followed by successive repetitions of that fixed cycle. Once the plateau is reached, increasing the number of repetitions does not affect the calculated error, indicating that stroboscopic sequence interrupts would be permitted without performance degradation. Beside providing a direct means of finding high-fidelity long-time DD schemes, these numerical results support our key analytic insights as to use of periodic sequence design. 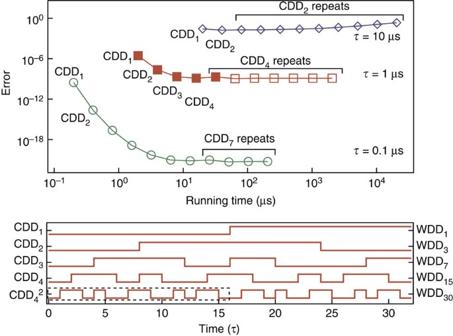Figure 3: Emergence of coherence plateau and sequence structure. Top: Minimal-error DD sequences from numerical search over Walsh DD, forτ=0.1, 1, 10 μs. In each series, the minimal-error sequences systematically access higher orders of error cancellation (via concatenation) over increasing running times, until an optimal concatenated sequence is found which is then repeated in the longer minimal-error sequences. The gradual increase in error (loss of plateau) for the series withτ=10 μs is due to the softness of the high-frequency cutoff and the constraints placed onTpby fixingτ. For the case ofτ=1 μs, we have calculated the error out tom≈108repeats (Ts≈103s, data not shown) without an observable effect from the soft cutoff. Bottom: Control propagators corresponding to the solid markers in the middle data series (τ=1 μs), showing the emergence of a periodic structure for sufficiently long-storage time. Labels indicate the corresponding sequence designations in either the CDD or Walsh basis. Control propagators scaled to same length for ease of comparison. Dashed box highlights base sequence CDD4that is repeated for long times. Figure 3: Emergence of coherence plateau and sequence structure. Top: Minimal-error DD sequences from numerical search over Walsh DD, for τ =0.1, 1, 10 μs. In each series, the minimal-error sequences systematically access higher orders of error cancellation (via concatenation) over increasing running times, until an optimal concatenated sequence is found which is then repeated in the longer minimal-error sequences. The gradual increase in error (loss of plateau) for the series with τ =10 μs is due to the softness of the high-frequency cutoff and the constraints placed on T p by fixing τ . For the case of τ =1 μs, we have calculated the error out to m ≈10 8 repeats ( T s ≈10 3 s, data not shown) without an observable effect from the soft cutoff. Bottom: Control propagators corresponding to the solid markers in the middle data series ( τ =1 μs), showing the emergence of a periodic structure for sufficiently long-storage time. Labels indicate the corresponding sequence designations in either the CDD or Walsh basis. Control propagators scaled to same length for ease of comparison. Dashed box highlights base sequence CDD 4 that is repeated for long times. Full size image Realistic effects For clarity, we have thus far relied on a variety of simplifications, including an assumption of pure phase decoherence and perfect π rotations. However, as we next show, our results hold in much less idealized scenarios of interest to experimentalists. We begin by considering realistic control limitations. Of greatest importance is the inclusion of errors due to finite pulse duration, as they will grow with T s if not appropriately compensated. Even starting from the dephasing-dominated scenario we consider, applying real DD pulses with duration τ π >0 introduces both dephasing and depolarization errors, the latter along, say, the y axis if control along x is used for pulsing. As a result, the conditions given in equation (3) can no longer guarantee a coherence plateau in general: simply incorporating ‘primitive’ uncorrected π -pulses into a high-order DD sequence may contribute a net depolarizing error substantial enough to make a plateau regime inaccessible. This intuition may be formalized, and new conditions for the emergence of a coherence plateau determined, by exploiting a generalized multi-axis FF formalism [35] , [40] , in which both environmental and finite-width errors may be accounted for, to the leading order, by adding in quadrature the z and y components of the ‘control vector’ that are generated in the non-ideal setting (see Methods). The end result of this procedure may be summarized in a transparent way: to the leading order, the total FF can be written as , where F p ( ω ) is the FF for the bang–bang DD sequence previously defined and F pul ( ω ) depends on the details of the pulse implementation. Corrections in the pre-factors A bb , A pul arise from higher-order contributions. The parameter α pul captures the error suppression properties of the pulses themselves, similar to the sequence order of error suppression α p . A primitive pulse results in α pul =1 due to the dominant uncorrected y -depolarization. An expression for the asymptotic DD error may then be obtained starting from equation (1) and separating . An additional constraint thus arises by requiring that both the original contribution of equation (2) and be finite. Thus, in order to maintain a coherence plateau in the long-time limit we now require We demonstrate the effects of pulse-width errors in Fig. 4c . When using primitive π x -pulses ( α pul =1), the depolarizing contribution due to F pul ( ω ) dominates the total value of . For the dephasing spectrum we consider, s =−2, the condition for maintenance of a plateau using primitive pulses is not met, and the total error grows unboundedly with m after a maximum plateau duration T max ≡ m max T p ( m max may be estimated by requiring that , along lines similar to those discussed in the Methods section). The unwanted depolarizing contribution can, however, by suppressed by appropriate choice of a higher-order ‘corrected’ pulse, such as a DCG [5] , [6] , already shown to provide efficient error suppression in the presence of non-Markovian time-dependent noise [35] . For a first-order DCG, the dominant error contribution is cancelled, resulting in α pul =2, as illustrated in Fig. 4a ; incorporating DCGs into the base DD sequence thus allows the coherence plateau to be restored. For small values of τ π , the error contribution remains small and the plateau error is very close to that obtained in the bang–bang limit. Increasing τ π leads this error contribution to grow, and the plateau saturates at a new higher value. 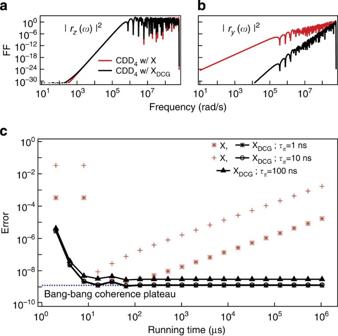Figure 4: Realistic FFs and effect of finite-width errors and soft cutoff. (a)z(dephasing) and (b)y(depolarization) quadrature components of the total FF for CDD4,F(ω)=Fp(ω)+Fpul(ω)≡|ry(ω)|2+|rz(ω)|2, incorporating non-zero duration uncorrectedπx-pulses (red), and first-order DCGs5,40,τπ=1 ns (see also Methods). In the ideal case, the depolarizing contribution |ry(ω)|2≡0, andF(ω)≡Fp(ω). The improvement of αpulfor CDD4with DCGs is demonstrated by the increased slope of |ry(ω)|2in panel (b). (c) DD error for theτ=1 μs data set ofFig. 3, using finite-duration pulses. Sub-Ohmic noise spectrum withs=−2 and soft Gaussian cutoff as inFig. 1are assumed. The low-value of αpulfor primitive pulses leads to unbounded error growth, terminating the plateau after a small number of repeats, determined by the ratio ofτπ/τ. Sequences incorporating DCGs meet the conditions for plateau out to at least 1 s storage time, with error increased by a factor of order unity compared with the bang–bang coherence plateau value, usingτπup to 100 ns. Outlier data points for CDD3arise because of even–odd effects in the FF when including pulse effects. Figure 4: Realistic FFs and effect of finite-width errors and soft cutoff. ( a ) z (dephasing) and ( b ) y (depolarization) quadrature components of the total FF for CDD 4 , F ( ω )= F p ( ω )+ F pul ( ω )≡| r y ( ω )| 2 +| r z ( ω )| 2 , incorporating non-zero duration uncorrected π x -pulses (red), and first-order DCGs [5] , [40] , τ π =1 ns (see also Methods). In the ideal case, the depolarizing contribution | r y ( ω )| 2 ≡0, and F ( ω )≡ F p ( ω ). The improvement of α pul for CDD 4 with DCGs is demonstrated by the increased slope of | r y ( ω )| 2 in panel ( b ). ( c ) DD error for the τ =1 μs data set of Fig. 3 , using finite-duration pulses. Sub-Ohmic noise spectrum with s =−2 and soft Gaussian cutoff as in Fig. 1 are assumed. The low-value of α pul for primitive pulses leads to unbounded error growth, terminating the plateau after a small number of repeats, determined by the ratio of τ π / τ . Sequences incorporating DCGs meet the conditions for plateau out to at least 1 s storage time, with error increased by a factor of order unity compared with the bang–bang coherence plateau value, using τ π up to 100 ns. Outlier data points for CDD 3 arise because of even–odd effects in the FF when including pulse effects. Full size image ‘Hardware-adapted’ DCGs additionally provide a means to ensure robustness against control imperfections (including rotation-angle and/or off-resonance errors) while incorporating realistic control constraints. For instance, sequences developed for singlet-triplet spin qubits [41] can simultaneously achieve insensitivity against nuclear-spin decoherence and charge noise in the exchange control fields, with inclusion of finite timing resolution and pulse rise times. A quantitative performance analysis may be carried out in principle through appropriate generalization of the FF formalism introduced above. Thus, the replacement of low-order primitive pulses with higher-order corrected pulses provides a straightforward path toward meeting the conditions for a coherence plateau with realistic DD sequences. These insights are also supported by recent DD nuclear magnetic resonance experiments [31] , [32] , that have demonstrated the ability to largely eliminate the effects of pulse imperfections in long pulse trains. Another experimentally realistic and important control imperfection is limited timing precision. The result of this form of error is either premature or delayed memory access at time T′ s = mT p ±δ t , offset relative to the intended one. Qualitatively, the performance degradation resulting from such access-timing errors may be expected to be similar to the one suffered by a high-order DD sequence under pulse-timing errors, analysed previously [24] . A rough sensitivity estimate may be obtained by adding an uncompensated ‘free-evolution’ period of duration δ t following the m th repeat of the sequence, with the resulting FF being determined accordingly. In this case, the effective order of suppression transitions α p →0, appropriate for free evolution, at a crossover frequency determined by the magnitude of the timing jitter. In order to guarantee the desired (plateau) fidelity level, it is necessary that the total FF—including timing errors—still meets the requirements set in equation (4). In general, this is achievable for supra-Ohmic spectra with s >1. When these conditions are not met, the resulting error can be much larger than the plateau value if the jitter is appreciable. Therefore, access timing places a constraint on a system designer to ensure that quantum memories are clocked with low-jitter, high-resolution systems. Considering the situation analysed in Fig. 3 with τ =1 μs and ~1.3 × 10 −9 , we estimate that access jitter of order 1.5 ps may be tolerated before the total measured error exceeds the bound of 2 . As current digital delay generators allow for sub-ps timing resolution and ps jitter, the requisite timing accuracy is nevertheless within reach with existing technologies. We next address different aspects of the assumed noise model. Consider first the assumption of a hard spectral cutoff in bounding the long-storage time error. If such an assumption is not obeyed (hence residual noise persists beyond ω c ), it is impossible to fully avoid the singular behaviour introduced by the periodic modulation as m →∞. Contributions from the resonating region ω ≈ ω res are amplified with m , and, similar to pulse-errors, cause to increase unboundedly with time and coherence to ultimately decay to zero. Nonetheless, a very large number of repetitions, m max , may still be applied before such contributions become important (note that this is the case in the previous figures, where we assume a soft Gaussian cutoff). We lower-bound m max by considering a scenario in which a plateau is preserved with a hard cutoff and estimating when contributions to error for frequencies ω > ω c become comparable to the plateau error. For simplicity, we assume that noise for ω > ω c falls in the passband of the FF and that at ω = ω c , the noise power-law changes from ω s → ω − r , with r >0. Treating such a case with s =−2 and using again repeated CDD 4 with τ =1 μs as in Fig. 3 , we find that as long as r is sufficiently large, the plateau error ~10 −9 can persist for m max 10 4 –10 6 repetitions (that is, up to a storage time of over 10 s), before the accumulated error due to high-frequency contributions exceeds the plateau coherence (see Methods). This makes it possible to engineer a coherence plateau over an intermediate range of T s , which can still be exceptionally long from a practical standpoint, depending on the specific rolloff behaviour of S ( ω ) at frequencies beyond ω c . Lastly, we turn to consideration of more general open-system models. For instance, consider a system–bath interaction, which includes both a dominant dephasing component and an ‘off-axis’ perturbation, resulting in energy relaxation with a characteristic time scale T 1 . Then the initial dephasing dynamics, including the onset of a coherence plateau, will not be appreciably modified so long as these two noise sources are uncorrelated and there is a sufficient separation of time scales. If , and the maximum error per cycle is kept sufficiently small, the plateau will persist until uncorrected T 1 errors dominate . We reiterate that in many experimentally relevant settings—notably, both trapped-ion and spin qubits— T 1 effects may indeed be neglected up to very long-storage times. Ultimately, stochastic error sources due, for instance, to spontaneous emission processes and/or Markovian noise (including white control noise) may form a limiting mechanism. In such circumstances, the unfavourable exponential scaling of Markovian errors with storage time poses a problem for high-fidelity storage through DD alone. Given a simple exponential decay with time-constant T M and assuming that equation (4) is met, we may estimate a maximum allowed plateau duration as . Thus, even with T M =100 s, a plateau at =10 −5 would terminate after T max =1 ms. Our results thus confirm that guaranteeing high-fidelity quantum memory through DD alone requires Markovian noise sources to be minimized, or else motivates the combination of our approach with quantum error correction protocols. The potential performance provided by our approach is quite remarkable. Besides the illustrative error calculations we have already presented, we find that many other interesting scenarios arise where extremely low-error rates can be achieved in realistic noise environments for leading quantum technologies. For instance, ytterbium ion qubits, of direct relevance to applications in quantum repeaters, could allow long-time, low-error coherence plateaus at the time scale of hours, based on bare free-induction-decay (1/ e ) times of order seconds [39] . Calculations using a common 1/ ω noise power spectrum with CDD 2 , a Gaussian high-frequency cutoff near 100 Hz, τ =1 ms and DCG operations with τ π =10 μs, give an estimate of the plateau error rate of 2.5 × 10 −9 . This kind of error rate—and the corresponding access latency of just 4 ms—has the potential to truly enable viable quantum memories for repeater applications. Similarly, the calculations shown throughout the manuscript rely on the well-characterized noise power spectrum associated with nuclear-spin fluctuations in spin qubits. Appropriate sequence construction and timing selection [41] permits the analytical criteria set out in equation (3) to be met, and similar error rates to be achieved, subject to the limits of Markovian noise processes as described above. In summary, we have addressed a fundamental and timely problem in quantum information processing—determining a means to effectively produce a practically useful high-fidelity quantum memory, by using dynamical error suppression techniques. We have identified the key requirements towards this end, and developed a strategy for sequence construction based on repetition of high-order DD base sequences. Our results allow analytical bounding of the long-time error rates and identify conditions in which a maximum error rate can be stroboscopically guaranteed for long times with small access latencies, even in the presence of limited control. We have validated these insights and analytic calculations using an efficient search over Walsh DD sequences assuming realistic noise spectra. The results of our numerical search bear similarity to an analytically defined strategy established in Hodgson et al . [27] for optimizing long-time storage in a supra-Ohmic excitonic qubit. From a practical perspective, our analyses help set technological targets on parameters such as error-per-pulse, timing resolution and Markovian noise strengths required to achieve the full benefits of our approach to quantum memory. This work also clearly shows how a system designer may calculate the impact of such imperfections for a specific platform, bound performance and examine technological trade-offs in attempting to reach a target memory fidelity and storage time. As the role of optimization in any particular setting is limited to finding a low-error sequence of duration T p to be repeated up to T s , our framework dramatically reduces the complexity of finding high-performance DD protocols. Future work will characterize the extent to which similar strategies may be employed to tackle more generic quantum memory scenarios. For instance, recent theoretical methods permit consideration of noise correlations across different spatial directions [40] in general non-Markovian single-qubit environments for which T 2 and T 1 may be comparable. In such cases, multi-axis DD sequences such as XY4 (ref. 2 ) may be considered from the outset in order to suppress phase and energy relaxation, as experimentally demonstrated recently [42] . Likewise, we remark that our approach naturally applies to multiple qubits subject to dephasing from independent environments. As expressions similar to the spectral overlap integral still determine the decay rates of different coherence elements [43] , exact DD can be achieved by simply replacing individual with collective π pulses, and conditions similar to equation (2) may then be separately envisioned to ensure that each coherence element saturates, again resulting in a guaranteed high-storage fidelity. Addressing the role of correlated dephasing noise and/or other realistic effects in multi-qubit long-time storage represents another important extension of this work. Inclusion of pulse errors Consider a base sequence p of total duration T p , including both free-evolution periods and control pulses with non-zero duration τ π , where the center of the j th pulse occurs at time t j ≡ δ j T p , with δ j [0, 1]. FFs that incorporate, to leading order in T p , errors due to both dephasing dynamics and non-ideal pulses are derived following [40] . The total FF, F ( ω )= F p ( ω )+ F pul ( ω ), may be expressed as where r z ( y ) are, respectively, the total z ( y ) components of the control vector for pure dephasing in the relevant quadrature, determined by the toggling-frame Hamiltonian associated with the control sequence. In the ideal bang–bang limit, , where for example, α p =4, for CDD 4 . In general, the total contributions to the FF are where and we incorporate pulse contributions through . For primitive pulses with a rectangular profile, and Ω≡ π / τ π , direct calculation yields [35] : For the three-segment first-order DCG we employ, one finds instead [35] , [40] : where . Starting from these expressions and suitably Taylor-expanding around ω =0, one may then show that the dominant pulse contributions arise from r y ( ω ) in the uncorrected case, with α pul =1 and A pul =− T p τ π /π, whereas they arise from r z ( ω ) in the DCG case, with α pul =2 and Assuming a noise power spectrum with a hard cutoff, S ( ω )= g ( ω / ω c ) s × Θ( ω − ω c ), the following expression for the (leading order) total asymptotic DD error, , is obtained: leading to the plateau conditions quoted in equation (4). Effect of a soft spectral cutoff Consider, again, a high-order DD sequence which is implemented with realistic pulses and is repeated m times. Then the leading contribution to the DD is given by where the FF F ( ω ) is computed as described above and S ( ω )= g ( ω / ω c ) s f ( ω , ω c ). While this integral converges nicely if we assume a sharp high-frequency cutoff, this is rarely encountered in reality. For a soft spectral cutoff, we can break the error integral up into two (low frequency versus high frequency) contributions, say, . We wish to estimate how many repeats of the base sequence are permitted under conditions otherwise leading to a plateau, before corrections due to the high-frequency tail dominate the error behaviour and destroy the plateau. Assume that the conditions given in equation (4) are obeyed, and let the maximum number of allowed repetitions be denoted by m max . Then m max may be determined by requiring that . As, for every m , we have , a lower bound for m max may be obtained by estimating m * such that . We may therefore simply identify with the hard-cutoff asymptotic value given in equation (9). In order to obtain an explicit expression for the high-frequency contribution, we assume that the noise power above ω c also takes a power-law form, S ( ω )= g ( ω / ω c ) r , formally corresponding to a rolloff f =( ω / ω c ) r − s , with power r >0. (Note that other possible choices of f , such as exponential or Gaussian rolloffs, may be treated along similar lines, at the expense of more complicated integrals). Thus, we may write where we have set the FF to the maximum value of the peaks in the passband. This value increases with pulse number and sequence order and must be calculated explicitly for a particular base sequence. For sufficiently large m , the oscillatory factor in the integrand may be approximated in terms of a Dirac comb, This allows us to write where we have exploited the fact that 0< ω c <2 π / T p and ζ( s ) denotes the Riemann zeta function. The error due to the soft rolloff at high frequencies thus increases linearly with m (hence T s = mT p ), as intuition suggests. As the zeta function is decreasing with r and attains its maximum value at r =0, corresponding to an infinite white noise floor, we obtain the following upper bound (recall that ζ(2)= π 2 /6): By equating and using Equations 9, 10, 11, 12, 13, 14, we finally arrive at the desired lower-bound: The above estimate can be applied, in particular, to the specific situation analysed in the main text: base sequence CDD 4 with τ =1 μs, DCG implementations with τ π ≤10 ns, and s =−2. In this case T p ≈16 μs, α p =4, , , and one can effectively neglect the contribution to m max due to pulse errors to within the accuracy of this lower bound. Let x ≡ T p ω c /2 π which, by the assumed plateau condition, ranges within [0,1]. Then we may rewrite implying that, for instance, at least 10 5 repetitions are allowed at x =0.001 if r ≥6, and at least 10 4 at x =0.01 if r ≥8. At the value x =0.16, corresponding to ω c /2π as used in the main text, r 18 ensures m max 10 4 hence a storage time of about T s ≈0.1 s with error as low as 10 −9 . As demonstrated by the data in Fig. 4 , T s is in fact in excess of 1 s under the assumed Gaussian cutoff, which is realistic for this system. In general, we have verified by direct numerical evaluation of the error integral in Equation (10) that, although qualitatively correct, the lower bound in Equation (16) can significantly under-estimate the achievable plateau length (for example, at x =0.16, a storage time T s ≈0.1 s is reached already at r 15). Altogether, this analysis thus indicates that high-frequency tails do not pose a practically significant limitation provided that the noise falls off sufficiently fast, as anticipated. How to cite this article: Khodjasteh, K. et al. Designing a practical high-fidelity long-time quantum memory. Nat. Commun. 4:2045 doi: 10.1038/ncomms3045 (2013).